A unified approach for divergent synthesis of contiguous stereodiads employing a small boronyl group Acyclic contiguous stereocenters are frequently seen in biologically active natural and synthetic molecules. Although various synthetic methods have been reported, predictable and unified approaches to all possible stereoisomers are rare, particularly for those containing non-reactive hydrocarbon substituents. Herein, a β -boronyl group is employed as a readily accessible handle for predictable α -functionalization of enolates with either syn or anti selectivity depending on reaction conditions. Contiguous tertiary-tertiary and tertiary-quaternary stereocenters are thus accessed in generally good yields and diastereoselectivity. Based on experimental and computational studies, mechanism for syn selective alkylation is proposed, and Bpin (pinacolatoboronyl) behaves as a smaller group than most carbon-centered groups. The synthetic utility of this methodology is demonstrated by preparation of several key intermediates for bioactive molecules. Introduction of substituents with predictable stereoselectivity is crucial for rational synthetic design of functional molecules. Despite the already advanced toolbox for practitioners of synthetic chemistry, it is still challenging to access any and every stereoisomer of contiguous acyclic stereodiads in a predictable fashion, particularly for substrates that contain only hydrocarbon groups [1] , [2] , [3] , [4] , [5] . For example, electrophilic α alkylation of an enolate is one of the most fundamental textbook transformation. [6] A venerable variant, Fráter–Seebach alkylation, can reliably produce the desired product with anti -selectivity ( I ) starting from β -hydroxyl carboxylate (Fig. 1a ) [7] , [8] , [9] . A cyclic lithium enolate intermediate involving chelation of the β -alkoxide anion is the key stereo-controlling factor. This method has been extensively employed in syntheses of polyketides and other natural products [10] , [11] . However, the syn -product III could not be obtained in similar vein (Fig. 1a ). Furthermore, when the β -substituent is a non-chelating group, usually no stereocontrol could be achieved (Fig. 1a , for II and IV ). Even in the extreme cases where R 1 could be a chiral auxiliary, it is still challenging to access both diastereomers ( II and IV ). Therefore, a unified approach for predictable construction of syn - and/or anti -stereodiads would be highly desirable yet, to the best of our knowledge, has remained elusive. Fig. 1: β -Controlled α -alkylation of carbonyl compounds. a Possible strategies in β -controlled construction of contiguous α , β -stereodiads. b Boronyl group-controlled unified approach to stereodiads via α -functionalization of β -boronyl esters. Full size image Considering that a boronyl group may be readily introduced by recent catalytic asymmetric borylation reactions [12] , [13] , [14] , [15] , [16] , [17] and could serve as a platform to access other functional groups in a stereospecific fashion [18] , [19] , [20] , [21] , [22] , [23] , [24] , [25] , [26] , we hope to develop a stereodivergent α -functionalizations of β -boronyl carbonyls with predictable diastereoselectivity employing the unique role of boronyl group (Fig. 1b ). The resulting acyclic compounds bearing contiguous tertiary–tertiary or even tertiary–quaternary stereogenic centers should have great value in syntheses of natural products and pharmaceuticals [27] , [28] , [29] , [30] . In the past few years, a number of catalytic approaches to boronyl-containing 1,2-stereodiads have been reported by Miura, Ito, Liao, Brown, and other groups [31] , [32] , [33] , [34] , [35] , [36] , [37] , [38] , [39] , [40] , [41] , [42] , [43] , [44] . However, usually only one diastereomer rather than the other is preferred, and development of general and reliable methodologies for obtaining all possible stereoisomers of β -boron carbonyls remains highly challenging [45] , [46] , [47] , [48] , [49] , [50] . The Ito group [51] and the Zhong group [52] have independently reported diastereoselective borylative alkylation of α , β -unsaturated esters. However, the enantioselective variant has not been accomplished. Herein, we wish to disclose our results in developing a practical and general, β -boronyl and conditions-controlled approach for divergent synthesis of both syn and anti -products containing contiguous tertiary–tertiary and tertiary–quaternary stereodiads (Fig. 1b ). Upon deprotonation, a cis -enolate (path A) or a trans enolate (path B) may be selectively generated. In the cis case, due to the Lewis acidic property of sp 2 boron atom, by invoking a five-membered chelation mode A , the anti -selectivity could be realized because the electrophile should attack from the less-hindered face of A (Fig. 1b ). On the other hand, if the deprotonation follows an Ireland model [53] , [54] , an open-chain trans intermediate B could be formed. 1,3-Allylic strain would induce a relatively fixed conformation and the facial selectivity of alkylation should be dictated by the relative size difference of the Bpin and R group (Fig. 1b , path B). Pleasingly, we discover that in all cases, the Bpin group behaves uniquely as a smaller group than R, and therefore the syn -product is generally favored. Reaction optimization We commenced the study by investigating the model reaction between β -boronyl esters 1a and allyl bromide 2 . 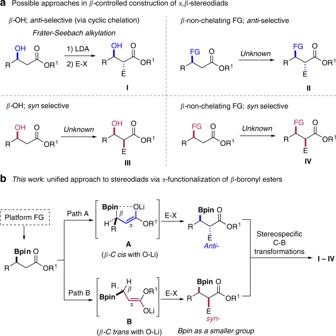Fig. 1:β-Controlledα-alkylation of carbonyl compounds. aPossible strategies inβ-controlled construction of contiguousα,β-stereodiads.bBoronyl group-controlled unified approach to stereodiads viaα-functionalization ofβ-boronyl esters. Simple treatment of a solution of 1a in THF with LDA (lithium diisopropylamide) followed by addition of 2 at −78 ° C led to a mixture of diastereomers favoring syn - 4a in 65% overall yield ( anti/syn = 1:2.4, Table 1 , entry 1). The relative configurations could be confirmed by transformation of the boronates to the corresponding alcohols. Although toluene was not an effective solvent for this reaction, a mixed solvents (THF/toluene = 1:1 v/v) could slightly improve the diastereoselectivity ( anti/syn = 1:3.9, Table 1 , entry 3). In contrast, when hexamethylphosphoramide (HMPA) was used as an additive, the anti -product 3a was obtained with excellent diastereoselectivity ( anti / syn > 20:1, Table 1 , entry 4), albeit in low yield (33%). Further, a modification of the ethyl ester 1a to 3-pentyl ester 1b markedly enhanced the syn -selectivity (Table 1 , entry 5, 77% yield, anti / syn = 1:10). A slightly higher syn -selectivity was achieved when some more toluene cosolvent was used (THF/toluene 1:1.5 v/v, Table 1 , entry 6). The best conditions for anti -product 3 was obtained when tert -butyl ester 1c was employed (Table 1 , entry 9, 75% yield, anti / syn > 20:1). Table 1 Condition optimization for the allylation of β- boronyl esters a . Full size table Substrate scope With optimal reaction conditions established, we explored the scope of these reactions. We found that the diastereodivergent reaction was successfully performed on a 2.0 mmol scale with little effects on the yield and selectivity (Figs. 2 , 3 c, 4b ). As shown in Fig. 2 , a variety of β -boronyl esters and electrophiles participated in these transformations in good to excellent yields with consistent diastereoselectivity for both syn and anti -products. For example, halide substituents on the aryl ring were well compatible in the reaction conditions ( 7a – 7c for anti and 8a – 8c for syn -products). The aromatic ring containing methoxy or trifluoromethoxy group proved to be competent reaction partners ( 7d , 7e , 8d , 8e ). It is noteworthy that, substrates with sterically demanding groups furnished the syn -products with higher diastereoselectivity when compared with the phenyl group ( 8f , 8g versus 4b ), which were consistent with our observation that Bpin served as the smaller group. The substrate bearing 2-thiophene furnished the syn -product with lower diastereoselectivity ( 8h , 62% yield, anti / syn = 1:2.5). This could be understood because the steric hindrance of 2-thiophenyl group should be smaller than phenyl group. Nevertheless, the anti -product 7 h was obtained with high diastereoselectivity. We next examined the viability of substrates with aliphatic substituents. To our surprise, the syn -product 8i could still be obtained with moderate selectivity ( anti/syn = 1:3.8), which means that Bpin behaves as a smaller group even than methyl group. As expected, the more bulkier alkyl group was employed, the higher syn -selectivity could be achieved ( 8j – 8n ). These results all pointed that Bpin acted as a smaller group in this transformation. In parallel, these β -boronyl esters containing aliphatic substituents successfully furnished the anti -products 7i – 7n with excellent diastereoselectivity. In addition, alkenyl-substituted β -boronyl esters also participated in this reaction and generated the corresponding products 7o – 7p and 8o – 8p with selectivity of same trend. Fig. 2: Substrate scope of the diastereodivergent α -functionalization of β -boronyl carbonyl compounds. Reaction conditions: unless otherwise noted, the reactions were performed at 0.25  mmol scale with 1.5 equiv allyl bromide, 1.1 equiv LDA, and 0.2 mL HMPA (if used). Isolated yields shown. D.r. values determined by 1 H NMR analysis of crude poducts. a Iodomethane as the electrophile. b Benzyl bromide as the electrophile. c Cinnamyl bromide as the electrophile. d Benzylchloromethyl ether as the electrophile. e 3-Bromo-1-(trimethylsilyl)-1-propyne as the electrophile. f Diphenyl disulfide as the electrophile. Full size image Fig. 3: Calculated free energy profiles for the α -alkylation of carbonyl compounds (R 1 = 3-pentyl). The favored pathway is labeled by solid lines. The values given in kcal/mol are the relative free energies calculated by the M06-2X/6-311 + G(d,p)//B3LYP/6-31 G(d) method in THF solvent. Full size image Fig. 4: Optimized structures at nucleophilic substitution steps. a Transition state of 9-ts and 11-ts . b Transition state of 9-ts-Me and 11-ts-Me . (R 1 = 3-pentyl). Full size image We also examined the scope with respect to other electrophiles. Beyond allyl substituent, methyl, benzyl, cinnamyl, benzyloxymethyl, and propargyl groups could also be installed to the β -boronyl esters with high selectivity for both syn and anti -products ( 7q – 7u and 8q – 8u ). Besides alkyls, the phenylthio group could also be introduced to the α -position of β -boronyl esters with excellent diastereoselectivity when diphenyl disulfide was employed as the electrophile ( 7v , 8v ). Finally, we tested similar alkylation of β -boronyl amides. However, only anti -products could be accessed under either set of conditions ( 7w – 7x ), probably because of the severe steric interaction between NEt 2 and β -carbon in the Ireland model, leading to exclusive formation of cis -enolate [55] . Mechanistic origins of the syn -selectivity Density functional M06-2X [56] with a standard 6-311 + G(d,p) basis set was employed to gain further insight into the diastereodivergent alkylation reactions, paticularly the general syn -selective outcome. In our theoretical calculations, the β -boryl ester 1 and allyl bromide 2 were chosen as reactants in model reaction, which can give syn -product 4b in experimental observations (Fig. 3 ). As depicted in Fig. 3 , ligand exchange between solvent-coordinated LDA C-3 and β -boryl ester 1 forms O-coordinated complex C-4 in an endothermic process with 4.0 kcal/mol free energy, which can attribute to the weak coordination ability of ester. In complex C-4 , the coordination onto lithium significantly increased the ester’s α -acidity. Subsequently, amino-assisted deprotonation of ester’s α -hydrogen can smoothly occur via either six-membered ring transition state 5-ts or 7-ts . The calculated relative free energy of 7-ts is 1.3 kcal/mol higher than that of 5-ts , indicating that the generation of open-chain enolate C-6 is favorable with 13.6 kcal/mol exergonic. The energy difference between transition states 5-ts and 7-ts can be attributed to the position of bulky boronylbenzyl group, which is located at the axial position in 7-ts . In this case, 1,3-allylic strain resulted in a lowest energy conformation, where the β -proton and the bulky ester group OR 1 of enolate C-6 are cis to each other and nearly coplanar [57] . The subsequent intermolecular nucleophilic substitution by enolate C-6 with allyl bromide 2 could occur through two different transition states owing to the chiral environment of β -C in enolate C-6 . The intermolecular nucleophilic substitution by the si -face of enolate C-6 onto the allyl bromide 2 could occur via linear transition state 9-ts , which leads to the generation of syn -product 4b from intermediate C-10 . On the contrary, the anti -isomer might be obtained via transition state 11-ts , where the nucleophilic substitution could take place by the re -face of enolate C-6 . The calculated energy barrier of transition state 11-ts is 12.9 kcal/mol, which is 1.9 kcal/mol higher than that of 9-ts . Therefore, the computational study depicted that the syn - 4b should be the major product, which is consistent with experimental observations. 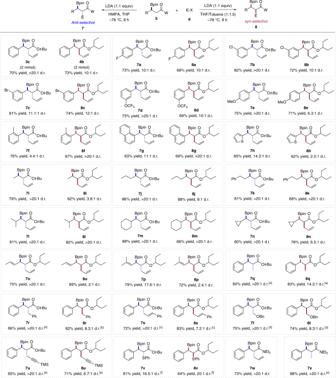Fig. 2: Substrate scope of the diastereodivergentα-functionalization ofβ-boronyl carbonyl compounds. Reaction conditions: unless otherwise noted, the reactions were performed at 0.25  mmol scale with 1.5 equiv allyl bromide, 1.1 equiv LDA, and 0.2 mL HMPA (if used). Isolated yields shown. D.r. values determined by1H NMR analysis of crude poducts.aIodomethane as the electrophile.bBenzyl bromide as the electrophile.cCinnamyl bromide as the electrophile.dBenzylchloromethyl ether as the electrophile.e3-Bromo-1-(trimethylsilyl)-1-propyne as the electrophile.fDiphenyl disulfide as the electrophile. As shown in Fig. 4a , optimized structure analysis shows that the main difference between 9-ts and 11-ts is the conformation of the α - and β -carbon atoms. To the satisfaction of the minimum steric repulsion of coming allyl bromide in nucleophilic substitution, the β -phenyl group and α -hydrogen adopt an eclipsed conformation in higher free energy transition state 11-ts , while, the β -boryl and α -hydrogen are eclipsed in transition state 9-ts . The phenyl group is larger than that of boryl group, which causes larger steric repulsion between eclipsed β -phenyl group and α -hydrogen in transition state 11-ts . Based on the aforementioned theoretical results, we hypothesized when the bulky phenyl group is masked by a smaller methyl group, poor diastereoselectivity will be observed in the experiment. As shown in Fig. 4b , in the nucleophilic substitution step, the calculated relative free energy of the re -face attack transition state 11-ts-Me is only 0.4 kcal/mol higher than that of si -face attack transition state 9-ts-Me . The theoretically calculated diastereoselectivity value for the methyl masked reaction would decrease to 2.8:1, which is consistent with the experimental observation value (3.8:1). Although the Bpin group contains a five-membered heterocycle and a bulky pinacol moiety, its planar structure combined with substituent-free oxygen atoms might render it a less sterically demanding structural unit than common carbon-centered groups. In a recent report, Tillin et al. also noted smaller size effect of Bpin in comparison with groups such as cyclohexyl [58] . Construction of tertiary–quaternary stereodiads The construction of quaternary carbon stereocenters, especially in an open-chain molecule, is usually a challenge in synthetic chemistry [59] . Encouraged by the above results, we proceeded with a second α -alkylation of the obtained products 7q and 3c under the standard anti -selective conditions. Pleasingly, the tertiary–quaternary diastereoisomers 9 and 10 were obtained with high stereoselectivity (Fig. 5 ). Therefore, all diastereoisomers of the tertiary–quaternary stereocenters could be obtained by simply changing the sequence of α -alkylation. In combination with the well-established enantioselective 1,4-borylation methods [12] , [13] , [14] , [15] , [16] , [17] , all possible stereoisomers could be accessed in such an approach. Fig. 5: Construction of tertiary–quaternary stereocenters. Preparation of the diastereoisomers 9 and 10 . Full size image Stereospecific C-B transformations To exemplify the versatility of this methodology in building contiguous stereodiads, we converted the organoboronic acid derivatives into other classes of compounds by using established methods (Fig. 6 ). For example, the diastereoisomeric diols 11 and 12 could be accessed easily by an oxidation–reduction sequence from 3c and 4b , respectively. Moreover, the hydroxymethylated product 13 could be prepared by using the in situ formed LiCH 2 Cl and subsequent oxidation with NaBO 3 [60] . Furthermore, the coupling of 2-lithiofuran with boronic ester 4b gave the arylated product 14 in high yield with complete stereoretention by using the protocol developed by the Aggarwal group [61] . Similarly, other heterocycles such as indole and furan groups could be installed without erosion in diastereomeric ratio. These 1,1-diaryl compounds are important pharmacophores, and their stereocontrolled preparation have been challenging through traditional protocols [62] , [63] , [64] , [65] . Fig. 6: Products Transformations. Transformations of the boronic ester to alcohols ( 11 and 12 ), hydroxymethyl ( 13 ), and heterocycles ( 14 , 15, and 16 ). Full size image In our previous work, the cis -diol 19 , a key intermediate of carbocyclic nucleosides [66] , was successfully employed for total synthesis of prostratin, a potent anti-HIV and antitumor natural product [67] . The trans -diol 22 is also an important synthetic intermediate of carbocyclic analogs of the antiviral ribavirin [68] . Evans aldol reaction was previously used for the synthesis of these diols. However, the use of stoichiometric amounts of chiral auxiliaries, excess expensive and sensitive Lewis acid n -Bu 2 BOTf limited the synthetic efficiency. Herein, based on the current approach, unified catalytic enantioselective syntheses of cis -diol 19 and trans -diol 22 can be achieved using inexpensive chmicals (Fig. 7 ). Optically pure 5o was obtained through Cu-catalyzed enantioselective 1,4-borylation of the sorbic acid-derived ester [69] , [70] . Diastereoselective α -allylation of chiral 5o with standard conditions and subsequent oxidation with NaBO 3 furnished 17 and 20 in good yields. The cis -diol 19 and trans -diol 22 were then obtained by ring-closing olefin metathesis of 17 and 20 followed by reduction with LiAlH 4 , respectively. Fig. 7: Synthetic utility of the divergent methodology. Unified enantioselective synthesis of cis and trans diols 19 and 22 . Full size image In conclusion, we have developed a predictable and unified protocol for both syn and anti diastereoselective α -functionalization of readily available β -boronyl carbonyls. The key to success was the exploitation of the dual roles of Bpin: its apparently small size and its Lewis acidic character. The structural predictability, operational simplicity, and broad substrate scope in combination with the versatile role of Bpin in synthetic transformations should render the method useful in preparation of contiguous diads, which are present in many types of biologically active molecules yet difficult to access by conventional approaches. The surprising size effect of a boronyl group may well be used in other parts of organoboron chemistry. General procedure for anti α -functionalized- β -boronyl esters A solution of diisopropylamine (0.275 mmol, 38.5 µL) in THF (0.5 mL) was cooled to 0 °C and treated with n -BuLi (110 µL, 2.5 M in hexane) dropwise. The reaction mixture was stirred for 15 min and cooled to −78 °C. To the freshly prepared solution of LDA, a solution was added of β -boronyl ester (0.25 mmol) in THF/HMPA (0.5 ml/0.2 ml) dropwise over 2 min. After stirring at the same temperature for 3 h, the electrophile (0.375 mmol) was added to the reaction mixture dropwise over 1 min and stirred for 8 h. Then the reaction was quenched with saturated aq. NH 4 Cl solution (1.0 mL) and diluted with DCM (5.0 mL). The layers were separated, the aqueous phase was extracted with DCM (2 × 5.0 mL), the combined organic phases were washed with water and brine, dried (MgSO 4 ) and concentrated in vacuo. The crude product was purified by flash column chromatography to yield the desired anti -product. General procedure for syn α -functionalized- β -boronyl esters A solution of diisopropylamine (0.275 mmol, 38.5 µL) in toluene (0.6 mL) was cooled to 0 °C and treated with n -BuLi (110 µL, 2.5 M in hexane) dropwise. 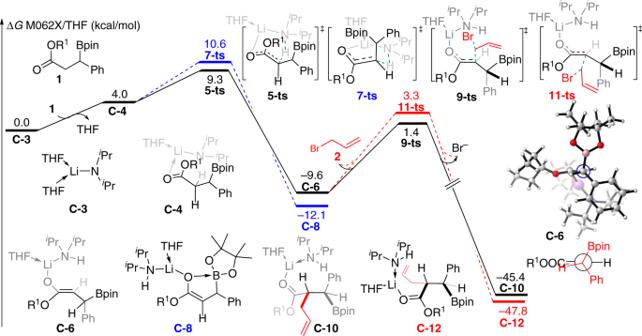Fig. 3: Calculated free energy profiles for theα-alkylation of carbonyl compounds (R1= 3-pentyl). The favored pathway is labeled by solid lines. The values given in kcal/mol are the relative free energies calculated by the M06-2X/6-311 + G(d,p)//B3LYP/6-31 G(d) method in THF solvent. The reaction mixture was stirred for 15 min and cooled to −78 °C. To the freshly prepared solution of LDA, a solution was added of β -boronyl ester (0.25 mmol) in THF (0.4 mL) dropwise over 2 min. After stirring at the same temperature for 15 min, the electrophile (0.375 mmol) was added to the reaction mixture dropwise over 1 min and stirred for 8 h. Then the reaction was quenched with saturated aq. NH 4 Cl solution (1.0 mL) and diluted with DCM (5.0 mL). 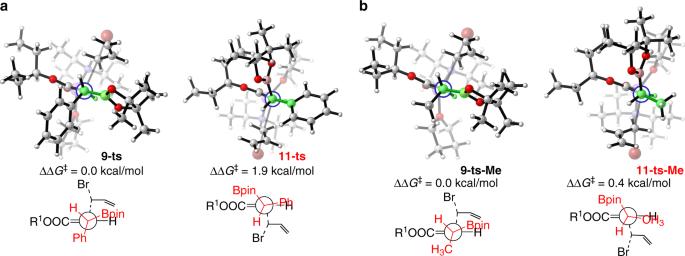Fig. 4: Optimized structures at nucleophilic substitution steps. aTransition state of9-tsand11-ts.bTransition state of9-ts-Meand11-ts-Me. (R1= 3-pentyl). The layers were separated, the aqueous phase was extracted with DCM (2 × 5.0 mL), the combined organic phases were washed with water and brine, dried (MgSO 4 ) and concentrated in vacuo. 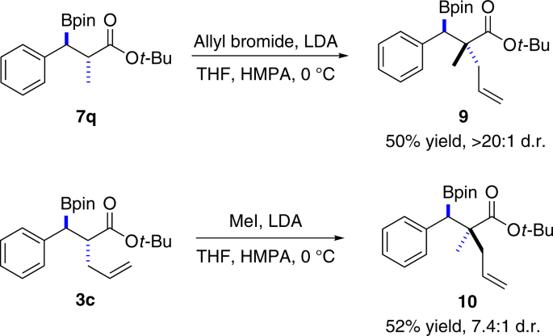Fig. 5: Construction of tertiary–quaternary stereocenters. Preparation of the diastereoisomers9and10. 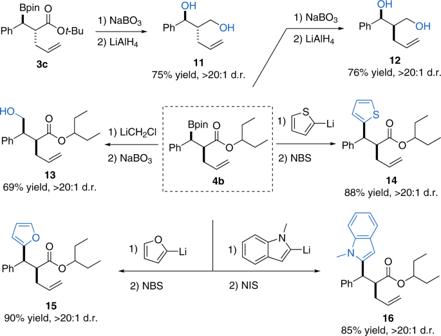Fig. 6: Products Transformations. Transformations of the boronic ester to alcohols (11and12), hydroxymethyl (13), and heterocycles (14,15,and16). 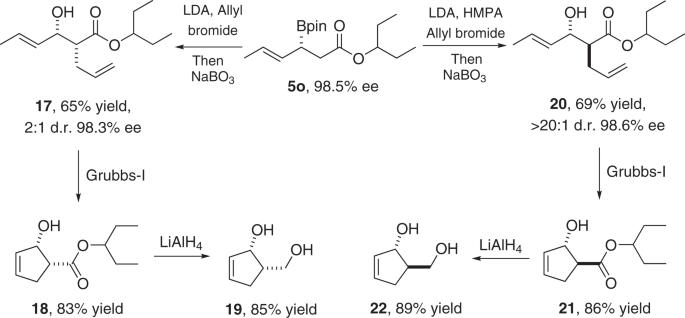Fig. 7: Synthetic utility of the divergent methodology. Unified enantioselective synthesis ofcisandtransdiols19and22. The crude product was purified by flash column chromatography to yield the desired syn -product. Spectroscopic methods 1 H NMR and 13 C NMR spectra were recorded using Bruker Avance 400 MHz spectrometers. High-resolution mass spectra (HRMS) were obtained on a WATERS I-Class VION IMS QTof spectrometer. Enantiomeric excesses (ee) were determined by chiral HPLC analysis using Waters 2489 Series chromatographs using a mixture of HPLC-grade hexane and isopropanol as eluent.